Fast ion transport for synthesis and stabilization ofβ-Zn4Sb3 Mobile ion-enabled phenomena make β -Zn 4 Sb 3 a promising material in terms of the re-entry phase instability behavior, mixed electronic ionic conduction, and thermoelectric performance. Here, we utilize the fast Zn 2+ migration under a sawtooth waveform electric field and a dynamical growth of 3-dimensional ionic conduction network to achieve ultra-fast synthesis of β -Zn 4 Sb 3 . Moreover, the interplay between the mobile ions, electric field, and temperature field gives rise to exquisite core-shell crystalline-amorphous microstructures that self-adaptively stabilize β -Zn 4 Sb 3 . Doping Cd or Ge on the Zn site as steric hindrance further stabilizes β -Zn 4 Sb 3 by restricting long-range Zn 2+ migration and extends the operation temperature range of high thermoelectric performance. These results provide insight into the development of mixed-conduction thermoelectric materials, batteries, and other functional materials. Mass transport, along with energy and charge transfer, is ubiquitous in nature and underscores diverse phenomena in science, engineering, and technology. Ionic migration is an important form of mass transport. On the one hand, electric field-driven ionic migration enables a wide range of applications such as batteries, fuel cells, and sensors [1] . On the other hand, ionic migration risks phase instability, for example, precipitation occurs when the mobile ion’s electrochemical potential is higher than its atomic counterpart. For the sake of phase stability, the voltage across an ionic conductor needs to be lower than the material-specific temperature-dependent threshold [2] . Here arise two profound questions. First, whether the mass transport in the form of ionic migration can be utilized towards fast materials synthesis. Mass transport mechanisms, different from the traditional thermal diffusion, are a frontier topic of materials science and engineering [3] . Second, whether the interplay between mobile ions, thermal, and electric fields can yield certain microstructures that stabilize the phase at a level beyond the aforementioned “threshold”. β -Zn 4 Sb 3 is a perfect material template to address these questions. β -Zn 4 Sb 3 is known for its complex crystal structure as well as the coexistence of mixed electronic and ionic conduction and promising thermoelectric (TE) performance in the low to intermediate temperature range (400–700 K) [4] , [5] , [6] , [7] , [8] , [9] , [10] , [11] , [12] , [13] . Unlike most state-of-the-art TE materials that are electron-based semiconductors or semimetals [14] , [15] , the mobile ions in β -Zn 4 Sb 3 play a vital role in its promising TE performance in the context of the Electron-Crystal Phonon-Liquid paradigm [16] . The weakly bonded Zn interstitials enable highly mobile Zn 2+ and also ultra-low thermal conductivity [17] , [18] , [19] , [20] . However, broader commercial applications of β -Zn 4 Sb 3 face two long-standing obstacles: developing time- and cost-efficient synthesis recipes and maintaining good phase stability [21] , [22] , [23] , [24] , [25] , [26] , [27] , [28] while delivering outstanding TE performance. To overcome these two β -Zn 4 Sb 3 -specific obstacles and to answer the two aforementioned general questions, here we have utilized the fast migration of Zn 2+ ions under electrical field and a dynamical growth of three-dimensional (3D) ionic conduction network to attain ultra-fast synthesis of β -Zn 4 Sb 3 . The presence of an electric field and the dynamic formation of 3D ionic conduction network speeded up the mass diffusion process and the chemical reaction of Zn and Sb into β -Zn 4 Sb 3 compared to the typical temperature-driven diffusion and chemical reactions. Due to the rapid cooling of the ion channel bulge when the current is cut off, the amorphous nonstoichiometric Zn 4 Sb 3 layer is formed and encapsulates crystalline β -Zn 4 Sb 3 grain. Such a core-shell crystalline-amorphous micromorphology, especially the amorphous grain boundary, restricts the migration of Zn 2+ ions across grains, and thus suppressed Zn precipitates. Hence, the as-formed core-shell microstructures self-adaptively suppress the thermodynamic re-entry instability of β -Zn 4 Sb 3 . Finally, doping by Cd or Ge on the Zn site as a steric hindrance further inhibits the migration of Zn 2+ ions within each grain. All these mechanisms worked jointly to improve the phase stability of β -Zn 4 Sb 3 and extend the operating temperature range of high TE performance. Fast synthesis Single-phase pristine β -Zn 4 Sb 3 was formed quickly through an electric field-assisted synthesis (EFAS) process. A schematic diagram of the EFAS apparatus is shown in Fig. 1a . The stoichiometric admixture of Zn and Sb powders was loaded into a graphite die, the inner wall of which was coated with a layer of BN to ensure that maximum current passed through the admixture rather than the die wall. A thermocouple was inserted into the admixture to measure the reaction temperature. The system is evacuated and maintained at a vacuum level ≤20 Pa. The (Zn 1 − x Cd x ) 4 Sb 3 ( x = 0.005, 0.01, and 0.015) and (Zn 1 − x Ge x ) 4 Sb 3 ( x = 0.0025, 0.005, and 0.0075) samples were synthesized under the same EFAS condition as pristine β -Zn 4 Sb 3 . Fig. 1: Ultra-fast synthesis, composition, and properties of β -Zn4Sb3-based materials. a Schematic diagram of the reaction apparatus, “1–4” represents the DC pulse power supply, graphite die, BN layer, stoichiometric admixture of Zn and Sb powders, respectively. b Time profile of the reaction parameters, including the loading pressure, temperature of the admixture, displacement of the graphite punch, current, voltage, and sintering function (i.e., the derivative of displacement). c Phase composition of the synthesized samples (standard XRD spectra of PDF#01-089-1969). d Room temperature electrical conductivity of MQ + SPS Zn 4 Sb 3 , EFAS Zn 4 Sb 3 , EFAS Zn 3.96 Cd 0.04 Sb 3 , and EFAS Zn 3.97 Ge 0.03 Sb 3 samples before and after a test cycle; “A” and “Z” represent the sample at the beginning and end of the electrical conductivity test. e Room temperature Zn 2+ ionic conductivities of MQ + SPS Zn 4 Sb 3 , EFAS Zn 4 Sb 3 , EFAS Zn 3.96 Cd 0.04 Sb 3 , and EFAS Zn 3.97 Ge 0.03 Sb 3 samples (orange arrow indicating the decline of ionic conductivity). 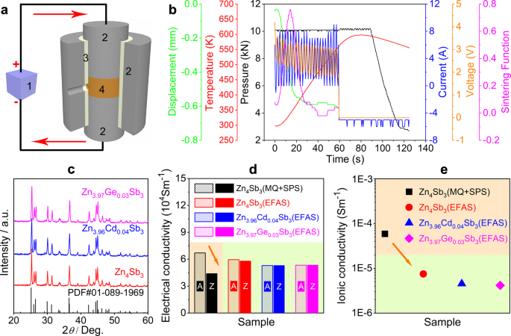Fig. 1: Ultra-fast synthesis, composition, and properties ofβ-Zn4Sb3-based materials. aSchematic diagram of the reaction apparatus, “1–4” represents the DC pulse power supply, graphite die, BN layer, stoichiometric admixture of Zn and Sb powders, respectively.bTime profile of the reaction parameters, including the loading pressure, temperature of the admixture, displacement of the graphite punch, current, voltage, and sintering function (i.e., the derivative of displacement).cPhase composition of the synthesized samples (standard XRD spectra of PDF#01-089-1969).dRoom temperature electrical conductivity of MQ + SPS Zn4Sb3, EFAS Zn4Sb3, EFAS Zn3.96Cd0.04Sb3, and EFAS Zn3.97Ge0.03Sb3samples before and after a test cycle; “A” and “Z” represent the sample at the beginning and end of the electrical conductivity test.eRoom temperature Zn2+ionic conductivities of MQ + SPS Zn4Sb3, EFAS Zn4Sb3, EFAS Zn3.96Cd0.04Sb3, and EFAS Zn3.97Ge0.03Sb3samples (orange arrow indicating the decline of ionic conductivity). Full size image Figure 1b displays the key reaction parameters, including the loading pressure, the temperature of the admixture, displacement of the graphite punch, current, voltage, and sintering function (i.e., the derivative of the displacement), as a function of time. The amplitude of current and voltage with a sawtooth waveform and a frequency of 0.4 HZ were applied in the range of 0–9 A and 1.8–3.6 V, respectively. The highest temperature measured during the passage of the current was 598 K, much lower than the growth-from-the-melt temperature of 1023 K [4] , [5] , and the SPS synthesis temperature of ~700 K [29] , [30] for β -Zn 4 Sb 3 based materials. At about 10 s after the current was on, the sintering function peaked, suggesting the onset of reaction. At ~20 s, the displacement of the graphite punch reached its maximum. After 60 s, Zn 4 Sb 3 , Zn 3.96 Cd 0.04 Sb 3 , and Zn 3.97 Ge 0.03 Sb 3 compounds were obtained with a relative density higher than 98%, as shown in Fig. 1c and Supplementary Figs. 1 and 2 . A reference pristine sample of β -Zn 4 Sb 3 was prepared using the melt-quench method followed by spark plasma sintering (hereafter named the MQ + SPS sample). The MQ + SPS sample was prepared from high purity elemental Zn shots (5N) and Sb chunks (5N), mixed and sealed in a silica tube under a pressure of 10 −3 Pa. The tube was slowly heated up to 1023 K and dwelt for 12 h, followed by quenching in saltwater. The obtained ingot was hand-ground into fine powders and consolidated using an SPS apparatus at 713 K for 4 min under a pressure of 30 MPa. The relative packing density of the as-prepared pellets, with a diameter of 16 mm and a thickness of 3 mm, was 97.6%. Supplementary Fig. 3 shows the phase composition of Zn 4 Sb 3 (MQ + SPS). The X-ray diffraction pattern confirmed the single-phased nature of β -Zn 4 Sb 3 (rhombohedral structure). Robust properties β -Zn 4 Sb 3 is a high-performance TE material made of cheap and relatively nontoxic elements. TE materials directly convert heat into electricity through the Seebeck effect, or function as heat pumps via the Peltier effect, thereby playing an important role in our global package of renewable energy options [14] , [15] . The efficiency of a TE material is gauged by its dimensionless figure of merit ZT , defined as ZT = α 2 σT /( κ L + κ e ), where α , σ , κ L , κ e , and T are the Seebeck coefficient, electrical conductivity, lattice thermal conductivity, electronic thermal conductivity, and the absolute temperature, respectively [14] , [15] . The detailed TE transport measurements of the Zn 4 Sb 3 -based samples were performed, as shown in Supplementary Figs. 4 – 12 . The EFAS Zn 4 Sb 3 -based compounds show excellent TE performance. For the EFAS Zn 3.96 Cd 0.04 Sb 3 sample, the maximum ZT value of 1.2 is achieved at 693 K (cf. Supplementary Fig. 7 ), while for the EFAS Zn 3.97 Ge 0.03 Sb 3 sample, the maximum ZT value of 1.12 is achieved at 700 K (cf. Supplementary Fig. 10 ). Upon doping with Cd or Ge, the overall ZT value increases in comparison with that of the pristine Zn 4 Sb 3 sample in the entire range of temperatures (cf. Supplementary Figs. 7 and 10 ). In history, the promising TE performance of β -Zn 4 Sb 3 -based compounds is overshadowed by the phase instability between 425 and 565 K [18] , and also the severe ion migration and Zn precipitates (kinetics instability) under an applied electric field even at room temperature (cf. Supplementary Fig. 13 ). For example, the MQ + SPS Zn 4 Sb 3 sample shows very different TE properties when measured twice, and the sample undergoes irreversible change during the measurement (cf. Supplementary Fig. 14 ). In contrast, the electrical conductivity, Seebeck coefficient, thermal conductivity, and calculated ZT curves of the EFAS Zn 4 Sb 3 -based compounds are very repeatable and reproducible (cf. Supplementary Figs. 15 – 20 ). The room temperature electrical conductivity of all the samples before and after a test cycle is presented in Fig. 1d . It is obvious that the electrical conductivity of the MQ + SPS Zn 4 Sb 3 sample decreased significantly from 6.7 × 10 4 to 4.4 × 10 4 Sm −1 , and that of EFAS Zn 4 Sb 3 sample decreased slightly from 5.9 × 10 4 to 5.8 × 10 4 Sm −1 , while that of EFAS Zn 3.96 Cd 0.04 Sb 3 sample and that of EFAS Zn 3.97 Ge 0.03 Sb 3 sample remain almost unchanged at about 5.3 × 10 4 to 5.4 × 10 4 Sm −1 , respectively. We also measured the Zn 2+ conductivity and ran endurance tests under high current density at elevated temperatures. We employed a direct-current (DC) polarization method with electron-blocking electrodes to isolate the ionic conduction by filtering out the electronic conduction [2] , [31] , [32] . Commercial zinc-loaded montmorillonite served as the electrodes. As shown in Supplementary Fig. 21 , the Zn 2+ migration rate is found to be 3.3 × 10 −3 Sm −1 at room temperature by the alternating-current (AC) electrochemical impedance spectroscopy (EIS) [33] , [34] , [35] , [36] . Solid-state Au|zinc-loaded montmorillonite|Zn 4 Sb 3 -based compounds|zinc-loaded montmorillonite|Au pseudo-galvanic cell was constructed (cf. Supplementary Fig. 22 ), in which all Zn 4 Sb 3 -based samples have a similar size of 8 × 8 × 1.3 mm 3 . When the output voltage is close to 10 V, which is the device limit, the current is reduced from 25 μA in the MQ + SPS Zn 4 Sb 3 , to 3.5 μA in the EFAS Zn 4 Sb 3 , to 1.9 μA in the EFAS Zn 3.96 Cd 0.04 Sb 3 , and finally to <1.9 μA in the EFAS Zn 3.97 Ge 0.03 Sb 3 , as shown in Supplementary Figs. 23 – 26 . The room temperature ionic conductivities of MQ + SPS Zn 4 Sb 3 , EFAS Zn 4 Sb 3 , EFAS Zn 3.96 Cd 0.04 Sb 3 , and EFAS Zn 3.97 Ge 0.03 Sb 3 samples were calculated to be 5.9 × 10 −5 , 7.5 × 10 −6 , 4.5 × 10 −6 , and 4.2 × 10 −6 Sm −1 , respectively (cf. Fig. 1e ). Hence, the Zn 2+ conductivity in the EFAS samples is suppressed by an order of magnitude compared to the MQ + SPS sample, which partially explains the observed improvement in the phase stability and the reproducibility of transport data. Doping Cd or Ge further enhanced the phase stability as evidenced by the results of electromigration tests conducted at a temperature of 473 K, a DC current density of 20 A/cm 2 , and a charging time of 24 h (cf. Supplementary Figs. 27 and 28 ). For comparison, the electromigration test was also carried out on the MQ + SPS sample under the same conditions. Supplementary Figs. 29 – 32 show the fracture surface morphology of typical samples after the electromigration tests. Obvious cracking and precipitation of Zn whiskers are observed on the MQ + SPS Zn 4 Sb 3 sample (cf. Supplementary Fig. 29 ). In contrast, the grain surface of the EFAS Zn 4 Sb 3 sample only becomes rough with no discernible precipitation of Zn (cf. Supplementary Fig. 30 ), and the grain surface of the EFAS Zn 3.96 Cd 0.04 Sb 3 sample is very clean with only a small number of microcracks (cf. Supplementary Fig. 31 ). Even better results are obtained with the EFAS Zn 3.97 Ge 0.03 Sb 3 sample, which shows no cracks but a clean surface (cf. Supplementary Fig. 32 ). The above results corroborate that the chemical stability of the EFAS samples is greatly improved. Combined with doping at the Zn sites, particularly doping with Ge, makes the EFAS samples exceptionally stable even under a high DC electric field. In the following sections, we will pinpoint the microscopic origins of the phase formation and the phase stability. Phase formation mechanism To pinpoint the phase formation mechanism of β -Zn 4 Sb 3 in the EFAS process, we first need to differentiate the effect of heating (nondirectional) and the effect of electric field (directional). Specially, we pay close attention to two specific aspects: Aspect #1 Temporal window of phase formation. Single phased β -Zn 4 Sb 3 can be obtained within 60 s under a pulsed DC field. However, when the charging time extends past 83 s (cf. Supplementary Fig. 33 ), it is observed that ZnSb forms at the upstream side of the sample, and Zn whiskers precipitate at the sample’s downstream side. We invert the die and the sample (turned upside down) and charge for 18 s (cf. Supplementary Fig. 34 ), the Zn and ZnSb are gone, and a homogeneous β -Zn 4 Sb 3 sample re-emerges. These observations corroborate that (i) the as-formed β -Zn 4 Sb 3 serves as a fast transport channel of Zn 2+ ions, and (ii) there is a temporal window for the phase formation of β -Zn 4 Sb 3 , beyond which the decomposition occurs in the presence of an electric current. Aspect #2 The process of phase formation. The phase formation of β -Zn 4 Sb 3 is the result of the competition between field-assisted phase formation and phase decomposition. 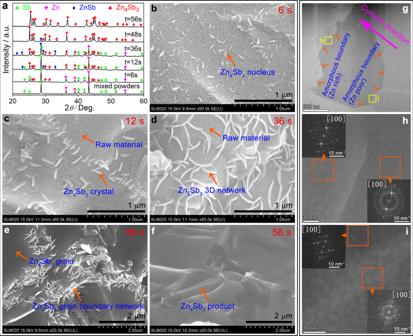Fig. 2: Phase transformation and microstructure evolution during the ultra-rapid synthesis ofβ-Zn4Sb3bulk material. aTemporal evolution of theβ-Zn4Sb3phase formation; microstructure transformation process ofβ-Zn4Sb3by FESEM:b6 s,c12 s,d36 s,e48 s,f56 s. Fine microstructure ofβ-Zn4Sb3by TEM:gmacroscopic image of grain,hmacroscopic image of grain boundary located at the downstream side of the current, and the illustration is the diffraction pattern in the orange frame area,imacroscopic image of grain boundary located at the upstream side of current, and the illustration is the diffraction pattern in the orange frame area. Figure 2a depicts a number of intermediate stages in the process of phase formation of β -Zn 4 Sb 3 . More detailed experimental results are provided in Supplementary Fig. 41 . When Zn and Sb powders are in physical contact, a small amount of β -Zn 4 Sb 3 is formed under the pulsed electric field within less than 10 s, the process is controlled by mutual inter-diffusion of Zn and Sb. Between 10 and 36 s, both the amount of ZnSb and β -Zn 4 Sb 3 increase simultaneously, as reflected by the peak in the sintering function curve in Fig. 1b . The appearance of ZnSb suggests that the transport speed of Zn 2+ ions is so fast in the ion channels of β -Zn 4 Sb 3 that Zn cannot be replenished in a timely manner so some are as-formed β -Zn 4 Sb 3 decomposes back into ZnSb and Zn. Then, the amount of ZnSb gradually decreases while that of β -Zn 4 Sb 3 further increases, which reflects the fact that the as-formed β -Zn 4 Sb 3 forms a 3D network and makes more Zn available to react with ZnSb into β -Zn 4 Sb 3 . Finally, β -Zn 4 Sb 3 is attained at the time of 56 s. Fig. 2: Phase transformation and microstructure evolution during the ultra-rapid synthesis of β -Zn 4 Sb 3 bulk material. a Temporal evolution of the β -Zn 4 Sb 3 phase formation; microstructure transformation process of β -Zn 4 Sb 3 by FESEM: b 6 s, c 12 s, d 36 s, e 48 s, f 56 s. Fine microstructure of β -Zn 4 Sb 3 by TEM: g macroscopic image of grain, h macroscopic image of grain boundary located at the downstream side of the current, and the illustration is the diffraction pattern in the orange frame area, i macroscopic image of grain boundary located at the upstream side of current, and the illustration is the diffraction pattern in the orange frame area. Full size image The microstructural evolution confirms that the as-formed β -Zn 4 Sb 3 serves as a fast transport channel of Zn 2+ ions, first form nuclei, and crystals, and then form a 3D network, through which Zn 2+ can be transported quickly under the electric field (cf. Figure 2b–f ). Finer microstructure details of β -Zn 4 Sb 3 were investigated by TEM (cf. Figure 2g–i ). The crystal grain shows a perfect β -Zn 4 Sb 3 lattice, while the grain boundary appears to be amorphous. The amorphous grain boundary located at the downstream side of current is rich in Zn (cf. Fig. 2h ), while the counterpart at the upstream side of current is poor in Zn (cf. Fig.e 2i ), de facto forming a special core-shell structure composite. These results point toward a schematic diagram of the reaction mechanism as shown in Fig. 3a–f . When Zn is in physical contact with Sb, under the pulse current, β -Zn 4 Sb 3 nucleus forms (cf. Fig. 3b ). Due to the high ionic conductivity of Zn 2+ in β -Zn 4 Sb 3 , Zn 2+ ions are easily transported through the as-formed β -Zn 4 Sb 3 and react with Sb forming additional β -Zn 4 Sb 3 in spite of Zn being separated from Sb by β -Zn 4 Sb 3 (cf. Fig. 3c ). Due to the transport speed of Zn 2+ in the ion channel of β -Zn 4 Sb 3 mismatches the local supply of fresh Zn, the upstream and downstream side of grain boundaries tend to be, respectively, poor and rich in Zn along the current direction. As β -Zn 4 Sb 3 crystals contact each other (at ~36 s), a 3D network is formed (cf. 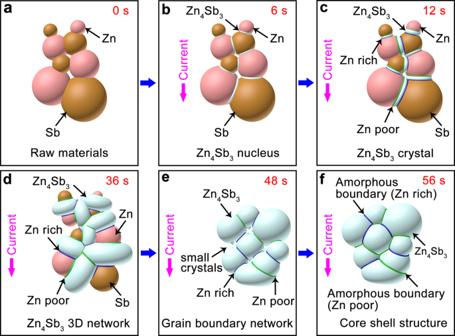Fig. 3: Schematic diagram of the reaction mechanism. aRaw materials of Zn and Sb powders with stoichiometric ratio.bβ-Zn4Sb3nuclei are formed at the contact point between Zn and Sb particles when the current is loaded (6 s).cβ-Zn4Sb3crystal grows up gradually, and the composition in the upstream region of the current is poor in Zn, while the composition in the downstream region is rich in Zn (12 s).dβ-Zn4Sb33D network is formed as growingβ-Zn4Sb3crystals contact each other (36 s).eSpecial grain boundary network structure filled with a large number ofβ-Zn4Sb3nanocrystals is formed due to the ion channel bulge.fCore-shell microstructure consisted of crystallineβ-Zn4Sb3grains and amorphous off-stoichiometric Zn4Sb3grain boundaries that are formed when the current is off. Figure 3d ), which greatly promotes the transport speed and scope of Zn 2+ ions and makes β -Zn 4 Sb 3 grains grow rapidly. In particular, a large number of β -Zn 4 Sb 3 nanocrystals are formed at the ion channel bulges, these nanocrystals fill the voids between Zn 4 Sb 3 grains, and lead to the densification of material (cf. Fig. 3e ). Normally, the current discharge at the grain boundary produces highly intensive Joule heating. When the current is off, the rapid cooling at the contact quenches nanocrystals to amorphous, forming the core-shell crystalline-amorphous microstructure (cf. Fig. 3f ). Fig. 3: Schematic diagram of the reaction mechanism. a Raw materials of Zn and Sb powders with stoichiometric ratio. b β -Zn 4 Sb 3 nuclei are formed at the contact point between Zn and Sb particles when the current is loaded (6 s). c β -Zn 4 Sb 3 crystal grows up gradually, and the composition in the upstream region of the current is poor in Zn, while the composition in the downstream region is rich in Zn (12 s). d β -Zn 4 Sb 3 3D network is formed as growing β -Zn 4 Sb 3 crystals contact each other (36 s). e Special grain boundary network structure filled with a large number of β -Zn 4 Sb 3 nanocrystals is formed due to the ion channel bulge. f Core-shell microstructure consisted of crystalline β -Zn 4 Sb 3 grains and amorphous off-stoichiometric Zn 4 Sb 3 grain boundaries that are formed when the current is off. Full size image Phase stability mechanism The core-shell crystalline-amorphous micromorphology somewhat explains the observed improvement of chemical stability of the EFAS samples because the amorphous layer is not ionic conducting. More details are provided by the in situ transmission electron microscopy study. The responses to an electric field applied to MQ + SPS Zn 4 Sb 3 sample and EFAS Zn 4 Sb 3 sample are recorded in detail in the Supporting information (cf. Supplementary Movies 1 and 2 ). In addition, Fig. 4a–f shows different stages (in time) when the current flows through the EFAS Zn 4 Sb 3 sample. When the applied voltage exceeds 0.69 V, the grain boundary is gradually widened, increasing from ~20 to ~74 nm, and, finally, the grain collapses and the material becomes unstable. 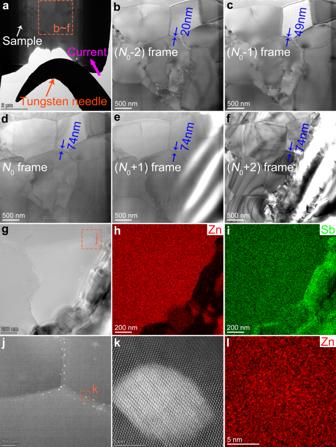Fig. 4: In situ microstructure evolution. a–fDifferent stages (in time) during the current flow through the EFAS Zn4Sb3sample (the grain boundary reaches the widest at theN0frame).g–iThe HAADF image and the corresponding EDS spectrum of EFAS Zn4Sb3sample after the current are turned off.jEnlarged HAADF image of the grain boundary area delineated by an orange border in (g); white particles are precipitated at the junction of the two grains.k–lHigh-resolution images and EDS spectra of white particles. Figure 4g–i shows the high-angle annular dark-field (HAADF) image and its corresponding energy-dispersive X-ray spectroscopy (EDS) spectrum of the EFAS Zn 4 Sb 3 sample after the current is turned off. It is obvious that the Zn 2+ ions migrate downstream along the current, and the upstream grains crack and fragment due to the loss of Zn. Fine structures of the grain boundary were studied (cf. Fig. 4j–l ). White particles, aka Zn metal, are precipitated at the junction of the two grains (cf. Fig. 4l ) and are amorphous (cf. Fig. 4k ). Interestingly, the surrounding areas of the white precipitates become crystalline. Apparently, when the applied voltage on the material is higher than the critical voltage, the amorphous grain boundary crystallizes into β -Zn 4 Sb 3 , which conducts Zn 2+ ions under the electric field and finally destabilizes the grain. On the contrary, as long as a voltage is applied, the grains of MQ + SPS Zn 4 Sb 3 sample will crack and disintegrate continually, and there is no phenomenon of grain boundary widening (cf. Supplementary Fig. 45 and Supplementary Movie 2 ). Fig. 4: In situ microstructure evolution. a – f Different stages (in time) during the current flow through the EFAS Zn 4 Sb 3 sample (the grain boundary reaches the widest at the N 0 frame). g – i The HAADF image and the corresponding EDS spectrum of EFAS Zn 4 Sb 3 sample after the current are turned off. j Enlarged HAADF image of the grain boundary area delineated by an orange border in ( g ); white particles are precipitated at the junction of the two grains. k – l High-resolution images and EDS spectra of white particles. 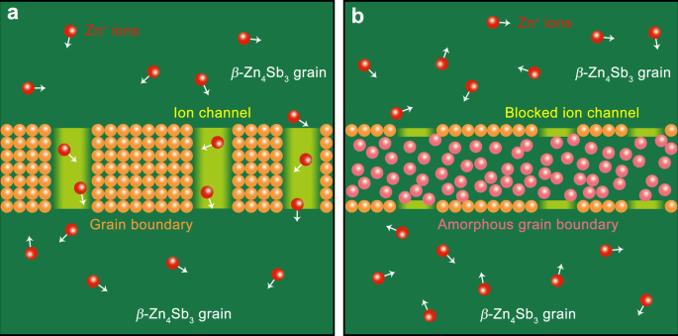Fig. 5: Ion blocking mechanism. aIon channels run through the grains to form a network all over the MQ + SPS Zn4Sb3bulk material.bIon channels in EFAS Zn4Sb3bulk material are limited to the interior of the grain, and the amorphous layer on the grain boundary (including rich Zn and poor Zn) blocks the formation of the network due to the lack of ion channel. Full size image Figure 5 shows the schematic diagram of β -Zn 4 Sb 3 microstructure derived by different synthesis methods. For MQ + SPS Zn 4 Sb 3 sample, ion channels run through the grains to the entire bulk as there is no ion migration blocking mechanism (cf. Fig. 5a ). While for the EFAS Zn 4 Sb 3 sample, ion channels are limited to the interior of the grain, and the amorphous layer on the grain boundary (respectively, poor and rich in Zn) blocks the formation of the network due to the lack of ion channels, so as to improve the stability of the bulk material (cf. Fig. 5b ). Moreover, the literatures [5] , [37] , [38] show that foreign elements can replace dynamic Zn, and thus reduce the ionic conduction and thus improve the stability. To sum up, the core-shell crystalline-amorphous microstructure combined with doping by foreign elements (i.e., Cd or Ge) at the Zn sites inhibit the migration of dynamic Zn 2+ ions at multiple scales, and improve the thermodynamic (phase transition, cf. Supplementary Figs. 43 and 44 ) and kinetic (ionic migration, cf. Supplementary Figs. 29 – 32 ) stability of β -Zn 4 Sb 3 . Fig. 5: Ion blocking mechanism. a Ion channels run through the grains to form a network all over the MQ + SPS Zn 4 Sb 3 bulk material. b Ion channels in EFAS Zn 4 Sb 3 bulk material are limited to the interior of the grain, and the amorphous layer on the grain boundary (including rich Zn and poor Zn) blocks the formation of the network due to the lack of ion channel. Full size image In summary, we have prepared a series of β -Zn 4 Sb 3 -based compounds with different dopants by an EFAS technique. The mechanism of phase formation and decomposition, and chemical stability, along with the TE transport properties, have been discussed in detail. Under the DC electric field, the ion transport channel in β -Zn 4 Sb 3 enables fast mass transport and participates in chemical reactions. A dense EFAS β -Zn 4 Sb 3 -based bulk material can be formed within 60 s. The resulting bulk composite material has a crystal-amorphous core-shell micromorphology. The as-formed composite microstructure, in conjunction with Cd/Ge doping, stabilizes the high TE performance of β -Zn 4 Sb 3 via suppressing the long-range Zn ions migration and precipitates of Zn on the grain boundaries. Specifically, the Zn 2+ ionic conductivity is decreased by more than an order magnitude from 5.9 × 10 −5 Sm −1 for the MQ + SPS sample to 4.2 × 10 −6 Sm −1 for the Ge-doped structure. Moreover, β -Zn 4 Sb was doped with 0.75 at.% Ge shows essentially no change when carrying the current density of 20 A/cm 2 at 473 K for 24 h. The Cd-doped structure Zn 3.96 Cd 0.04 Sb 3 attained ZT max = 1.2, at 693 K, while the Ge-doped Zn 3.97 Ge 0.03 Sb 3 sample reached ZT max = 1.12, at 700 K. The synthesis method can be in principle extended to, for example, ZnSb, Cu 2 Se, and Cu 2 S (cf. Supplementary Figs. 46 – 48 ), which is of great technical implications. Synthesis Four grams of Zn (5N, 200 mesh) and Sb (5N, 200 mesh) or Cd (5N, 200 mesh) and Ge (5N, 200 mesh) powders were weighed according to the stoichiometric ratio and were thoroughly mixed in an agate mortar for 20 min. The mixed raw powders were transferred into the mold (Φ16 mm) in Fig. 1a . The inner wall of the graphite mold was coated by a layer of BN to ensure most current flows through the powder admixture. A thermocouple was inserted into the admixture to measure the reaction temperature. In a typical process, a vacuum level ≤ 20 Pa was maintained. Next, a pulsed sawtooth-shaped current is applied to the mold for 60 s. The resulting pellet with a diameter of 16 mm and a height of 3 mm had a relative density of more than 98%. The ingot was cut into appropriate shapes for the TE property measurements and electromigration tests. Moreover, the EFAS processes for Bi 2 Te 3 , ZnSb, Cu 2 Se, and Cu 2 S compounds are really similar. Test of ionic conductivity of Zn 2+ The migration rate of Zn 2+ ions in the commercial zinc-loaded montmorillonite was tested through AC EIS. A solid-state Au|zinc-loaded montmorillonite|Zn 4 Sb 3 -based compounds|zinc-loaded montmorillonite|Au pseudo-galvanic cell was constructed, in which all Zn 4 Sb 3 -based samples have a similar size of 8 × 8 × 1.3 mm 3 . Then, based on the DC polarization measurements, the resulting ionic conductivities of Zn 4 Sb 3 (MQ + SPS), Zn 4 Sb 3 (EFAS), Zn 3.96 Cd 0.04 Sb 3 (EFAS), and Zn 3.97 Ge 0.03 Sb 3 (EFAS) at room temperature could be obtained. Chemical electromigration tests Electromigration tests were conducted at a temperature of 473 K, with the DC current density of 20 A/cm 2 , and the charging time of 24 h. High-purity argon gas of 100 Pa filled the cavity to avoid a short circuit. Characterization The phase purity of all samples was inspected by X-ray powder diffraction (Empyrean, Cu K α line, PANalytical, Holland). Images of freshly fractured surfaces were taken by field emission scanning electron microscopy (SU8000, Hitachi, Japan) with EDS (XFlash6160, Bruker, Germany). Back-scattered images were taken by EPMA (JXA-8100, JEOL, Japan). A direct characterization of the samples’ atomic structures and structural evolution during the process of electrification was carried out on transmission electron microscopy (Talos F200s, FEI) and double spherical aberration-corrected transmission electron microscopy (Titan Themis G2 60-300, FEI). The samples for TEM observation were prepared by ion milling with liquid nitrogen (PIPS 695, Gatan) and focused ion beam milling (Helios Nanolab G3 UC, FEI). In situ biasing experiments were performed within the TEM column using a TEM-STM holder (Pico Femto, Zeptools). The low- and high-temperature heat flow of the Zn 4 Sb 3 -based samples, respectively, was detected by Q2000 (TA, USA). The electrical conductivity ( σ ) and the Seebeck coefficient ( α ) were measured simultaneously using a commercial equipment (ZEM-3, Ulvac, Japan). The high-temperature Hall coefficient ( R H ) was measured in a magnetic performance testing system (NYMS, China), using the van der Pauw method under a reversible magnetic field of 1.5 T. The low-temperature σ and R H between 10 and 300 K were measured on a Physical Properties Measurement System (PPMS-9, Quantum Design, USA). The effective carrier concentration ( n H ) was calculated by the formula: n H = 1/ eR H , where e is the electron charge. The Hall mobility follows from μ H = σR H . The thermal conductivity was calculated from the relation κ = D × c p × ρ , where D is the thermal diffusivity coefficient, c p is the specific heat capacity, and ρ is the bulk density. D was measured using an LFA457 (Netzsch, Germany) laser flash apparatus. c p was taken as the Dulong–Petit law value. ρ was obtained by the Archimedes method.